ALKBH4-dependent demethylation of actin regulates actomyosin dynamics Regulation of actomyosin dynamics by post-transcriptional modifications in cytoplasmic actin is still poorly understood. Here we demonstrate that dioxygenase ALKBH4-mediated demethylation of a monomethylated site in actin (K84me1) regulates actin–myosin interaction and actomyosin-dependent processes such as cytokinesis and cell migration. ALKBH4-deficient cells display elevated K84me1 levels. Non-muscle myosin II only interacts with unmethylated actin and its proper recruitment to and interaction with actin depend on ALKBH4. ALKBH4 co-localizes with the actomyosin-based contractile ring and midbody via association with methylated actin. ALKBH4-mediated regulation of actomyosin dynamics is completely dependent on its catalytic activity. Disorganization of cleavage furrow components and multinucleation associated with ALKBH4 deficiency can all be restored by reconstitution with wild-type but not catalytically inactive ALKBH4. Similar to actin and myosin knock-out mice, homozygous Alkbh4 mutant mice display early embryonic lethality. These findings imply that ALKBH4-dependent actin demethylation regulates actomyosin function by promoting actin-non-muscle myosin II interaction. Actin is one of the most abundant proteins in eukaryotic cells. It exists both as monomeric (G-actin) and filamentous (F-actin) actin, and the switch between these two states is highly dynamic. Dynamic actin filament networks are involved in a large variety of cellular functions, including lamellipodium formation, cell motility and cytokinesis [1] . The actin networks are maintained through coordinated actions of a large number of regulatory proteins that modulate filament assembly and disassembly, as well as through contractility driven by myosin II motor proteins [2] , [3] . The process of defining the plane and position of the cleavage furrow during cytokinesis requires communication between microtubules and the actin cortex and it eventually results in F-actin and NM II assembling into the contractile ring [4] , [5] . The contractile ring is a highly dynamic structure with a rapid turnover of both F-actin and NM II (refs 6 , 7 ). Accumulation of F-actin in the contractile ring may occur by nucleation in the furrow or by transport of pre-existing actin filaments nucleated elsewhere [8] , [9] . NM II is the major motor protein involved in cytokinesis and its movement along F-actin as well as F-actin depolymerization is required for furrow ingression [10] , [11] . Various post-translational modifications (PTMs) have been identified in actin, including N-terminal arginylation, acetylated aspartate residues, phosphorylated tyrosine residues, and methylated histidine and lysine residues [12] , [13] , [14] , [15] , [16] . However, how these actin PTMs are involved in the regulation of actomyosin dynamics remains largely unknown. The superfamily of Fe(II) and 2-oxoglutarate (2OG, α-ketoglutarate)-dependent dioxygenases (PF03171) belongs to the non-heme iron protein family, which can hydroxylate inactivated C-H groups. This class of enzymes can catalyse the demethylation of a variety of substrates [17] , [18] . In E. coli , the Fe(II)/2OG dioxygenase AlkB catalyses demethylation of various types of methyl modified DNA bases following exposure to methylating agents [19] , [20] . Based on sequence homology within the catalytic domain of E. coli AlkB, 9 human AlkB homologs have been identified, ALKBH1-8 and the somewhat less conserved FTO (refs 21 , 22 ). Like E. coli AlkB, ALKBH2 and ALKBH3 have been shown to possess DNA repair activity in vivo [23] . We have recently demonstrated that FTO and ALKBH5 are RNA m 6 A (N 6 -methyl-adenosine) demethylases [24] , [25] . Demethylation of m 6 A appears to be involved in energy homeostasis and implies important roles for FTO and ALKBH5 in obesity, type II diabetes and fertility [25] , [26] , [27] , [28] , [29] . The AlkB domain of ALKBH8 has been shown to hydroxylate modified uridine in the wobble-position of certain tRNA isoacceptors [30] , [31] . ALKBH1 is the first human AlkB homologue shown to hydroxylate proteins. Like the S. pombe homologue, ALKBH1 catalyses demethylation of histone H2A in vivo and has been proposed to be involved in neural differentiation [32] , [33] . These findings suggest a very wide functional diversity of mammalian AlkB proteins, with substrates ranging from DNA and RNA to protein. Although ALKBH4 has been demonstrated to decarboxylate 2OG in vitro [34] , its substrate and biological function in mammalian cells are currently unknown. In the present study, we show that ALKBH4 mediates demethylation of actin K84me1 and thereby regulates the actin–myosin II interaction. In addition, we demonstrate that deletion of ALKBH4 is embryonically lethal and depletion leads to defects in cytokinesis and cell motility. Deletion of Alkbh4 causes embryonic lethality in mice To investigate the biological function of ALKBH4, we generated conditional Alkbh4 gene-targeted mice with LoxP sites flanking exons 2 and 3 of the endogenous Alkbh4 locus. These exons includes conserved residues presumed to constitute the Fe(II)-binding cluster and residues required for binding to the 5-carboxylate of the 2-oxoglutarate co-substrate [35] , [36] ( Fig. 1a and Supplementary Fig. S1a ). The resultant Alkbh4 +/L ( L refers to the floxed allele) mice were crossed with mice ubiquitously expressing Cre-recombinase to generate the Alkbh4 null allele ( Alkbh4 − ) ( Supplementary Fig. S1a–c ). Heterozygous Alkbh4 +/L and Alkbh4 +/− mice develop normally, with no apparent phenotype. However, Alkbh4 +/− intercrosses failed to give rise to homozygous Alkbh4 −/− offspring, and the Mendelian distribution between wild-type (WT) and heterozygous genotypes indicated that disruption of Alkbh4 results in embryonic lethality ( Fig. 1b ). 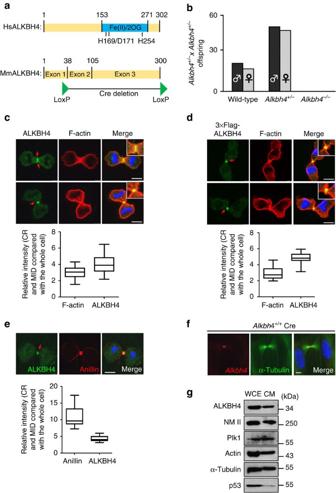Figure 1: Deletion of Alkbh4 causes embryonic lethality in mice and ALKBH4 associates with the contractile ring and midbody. (a) Schematic diagram showing human (upper panel) and mouse (lower panel) ALKBH4 protein structure with conserved catalytic amino acids within the dioxygenase domain (upper panel) and deleted exons in theAlkbh4knock-out allele (lower panel). (b) There were no homozygousAlkbh4−/−offspring from heterozygousAlkbh4+/−intercrosses. Mendelian distribution of WT and knock-out alleles indicated by the ratio 1:2:(1), WT: Het:(KO). +: WT allele; −: knock-out allele. (c) Endogenous ALKBH4 immunostaining in MRC5 cells with anti-ALKBH4 and F-actin staining with phalloidin. DNA was visualized by DAPI. Scale bars, 10 μm. Quantification of signal intensity (accumulation of protein) on the contractile ring (CR) and midbody (MID) relative to the whole cell (lower panel). (50 cells per condition per experiment). In box-and-whisker plot plotted by Prism5 software, median means 50% of cells is greater than this value, upper quartile or lower quartile means 25% cells is greater or less than this value and maximum or minimum means greatest or least value. (d) MRC5 cells stably expressing 3 × Flag-ALKBH4 were fixed and immunostained with anti-Flag and Phalloidin (F-actin). DNA was visualized by DAPI. Scale bars, 10 μm. Quantification of signal intensity (accumulation of protein) on the contractile ring (CR) and midbody (MID) relative to the whole cell (lower panel). (50 cells per condition per experiment). (e) MRC5 cells were fixed and immunostained with anti-ALKBH4 and anti-anillin (midbody marker). DNA was visualized by DAPI. Scale bars, 10 μm. Quantification of signal intensity (accumulation of protein) on the contractile ring (CR) and midbody (MID) relative to the whole cell (lower panel). (50 cells per condition per experiment). (f) MEF cells were fixed and immunostained with antibodies against ALKBH4 and α-tubulin (α-tub). DNA was visualized by DAPI. (g) MRC5 cells were sequentially synchronized with thymidine and nocodazole; and whole-cell extracts (WCE) and contractile ring/midbody (CM) fractions were analysed by immunoblotting with the indicated antibodies. Full-length blots are presented inSupplementary Fig. S7. Scale bars in all panels, 10 μm. Figure 1: Deletion of Alkbh4 causes embryonic lethality in mice and ALKBH4 associates with the contractile ring and midbody. ( a ) Schematic diagram showing human (upper panel) and mouse (lower panel) ALKBH4 protein structure with conserved catalytic amino acids within the dioxygenase domain (upper panel) and deleted exons in the Alkbh4 knock-out allele (lower panel). ( b ) There were no homozygous Alkbh4 −/− offspring from heterozygous Alkbh4 +/− intercrosses. Mendelian distribution of WT and knock-out alleles indicated by the ratio 1:2:(1), WT: Het:(KO). +: WT allele; −: knock-out allele. ( c ) Endogenous ALKBH4 immunostaining in MRC5 cells with anti-ALKBH4 and F-actin staining with phalloidin. DNA was visualized by DAPI. Scale bars, 10 μm. Quantification of signal intensity (accumulation of protein) on the contractile ring (CR) and midbody (MID) relative to the whole cell (lower panel). (50 cells per condition per experiment). In box-and-whisker plot plotted by Prism5 software, median means 50% of cells is greater than this value, upper quartile or lower quartile means 25% cells is greater or less than this value and maximum or minimum means greatest or least value. ( d ) MRC5 cells stably expressing 3 × Flag-ALKBH4 were fixed and immunostained with anti-Flag and Phalloidin (F-actin). DNA was visualized by DAPI. Scale bars, 10 μm. Quantification of signal intensity (accumulation of protein) on the contractile ring (CR) and midbody (MID) relative to the whole cell (lower panel). (50 cells per condition per experiment). ( e ) MRC5 cells were fixed and immunostained with anti-ALKBH4 and anti-anillin (midbody marker). DNA was visualized by DAPI. Scale bars, 10 μm. Quantification of signal intensity (accumulation of protein) on the contractile ring (CR) and midbody (MID) relative to the whole cell (lower panel). (50 cells per condition per experiment). ( f ) MEF cells were fixed and immunostained with antibodies against ALKBH4 and α-tubulin (α-tub). DNA was visualized by DAPI. ( g ) MRC5 cells were sequentially synchronized with thymidine and nocodazole; and whole-cell extracts (WCE) and contractile ring/midbody (CM) fractions were analysed by immunoblotting with the indicated antibodies. Full-length blots are presented in Supplementary Fig. S7 . Scale bars in all panels, 10 μm. Full size image ALKBH4 associates with the contractile ring and midbody Interestingly, immunofluorescence microscopy, using ALKBH4 antibodies generated for this study ( Supplementary Fig. S1d,e ) revealed a pronounced accumulation of ALKBH4 at contractile ring and midbody structures, as determined by co-localization of endogenous or overexpressed ALKBH4 with the contractile ring/midbody component F-actin ( Fig. 1c ) and anillin, an actomyosin scaffold protein and cleavage furrow marker ( Fig. 1e ). This staining pattern was also observed in Alkbh4 +/+ Cre mouse embryonic fibroblast (MEF) cells ( Fig. 1f ). Consistent with the immunofluorescence analysis, purification of contractile ring and midbody structures from human MRC5 cells demonstrated that a pool of ALKBH4 co-fractionated with the contractile ring and midbody proteins NM II, actin, α-tubulin and Plk1 ( Fig. 1g ). Taken together, these data suggest that ALKBH4 could be a novel factor involved in cytokinesis. This was further substantiated by mass spectrometric analysis of affinity-purified Flag-GFP-ALKBH4 protein complexes identifying the two key components of the actomyosin-based contractile ring, actin and NM II ( Supplementary Fig. S2a and Supplementary Table S1 ). These interactions were confirmed by endogenous and exogenous co-immunoprecipitation of ALKBH4 and actin or NM II ( Fig. 2a ), suggesting that ALKBH4 indeed is a bona fide component of the actomyosin network. Furthermore, the fact that incubation with magnesium and ATP prevents co-precipitation of NM II with ALKBH4 implies that the interaction between ALKBH4 and NM II is mediated by actin ( Fig. 2a ). 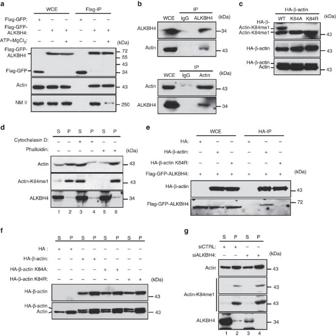Figure 2: Interaction of ALKBH4 with the actomyosin network and identification of actin K84 monomethylation. (a) Association between Flag-GFP-ALKBH4 and NM II assessed in 293T cells by immunoprecipitation. 293T cells were transfected with Flag-GFPor Flag-GFP-ALKBH4 constructs as indicated and lyisted in NET buffer, which didn’t contain EDTA. In all, 2 mM ATP and 2 mM MgCl2were added into NET buffer freshly. WCE, whole-cell extract. (b) Association between endogenous ALKBH4 and actin assessed in MRC5 cells by co-immunoprecipitation analysis of ALKBH4 and actin using indicated antibodies. (c) WCEs from 293T cells transfected with HA-β-actin WT, K84A or K84R were immunoblotted with the indicated antibodies. (d) Detection of free and filamentous actin by actin fractionation. Semi-confluent 293T cells were treated with or without 1 μg ml−1CCD and 1 μg ml−1phalloidin for 30 min at 37 °C as indicated. Soluble free G-actin (S) and insoluble filamentous F-actin (P). (e) 293T cells were co-transfected with Flag-GFP-ALKBH4 either WT or K84R HA-β-actin as indicated and lysates were subjected to HA immunoprecipitation. Immunoprecipitates and WCE were immunoblotted with the indicated antibodies. (f) Forty-eight hours after transfection with the indicated DNA constructs, 293T cells were lysed and subjected to F-actin fractionation. Fractions were analysed by immunoblotting with the indicated antibodies. (g) Forty-eight hours after transfection with the indicated siRNAs, 293T cells were lysed and subjected to F-actin fractionation assay. Fractions were analysed by immunoblotting with the indicated antibodies. Full-length blots in all panels are presented inSupplementary Fig. S7. Figure 2: Interaction of ALKBH4 with the actomyosin network and identification of actin K84 monomethylation. ( a ) Association between Flag-GFP-ALKBH4 and NM II assessed in 293T cells by immunoprecipitation. 293T cells were transfected with Flag-GFPor Flag-GFP-ALKBH4 constructs as indicated and lyisted in NET buffer, which didn’t contain EDTA. In all, 2 mM ATP and 2 mM MgCl 2 were added into NET buffer freshly. WCE, whole-cell extract. ( b ) Association between endogenous ALKBH4 and actin assessed in MRC5 cells by co-immunoprecipitation analysis of ALKBH4 and actin using indicated antibodies. ( c ) WCEs from 293T cells transfected with HA-β-actin WT, K84A or K84R were immunoblotted with the indicated antibodies. ( d ) Detection of free and filamentous actin by actin fractionation. Semi-confluent 293T cells were treated with or without 1 μg ml −1 CCD and 1 μg ml −1 phalloidin for 30 min at 37 °C as indicated. Soluble free G-actin (S) and insoluble filamentous F-actin (P). ( e ) 293T cells were co-transfected with Flag-GFP-ALKBH4 either WT or K84R HA-β-actin as indicated and lysates were subjected to HA immunoprecipitation. Immunoprecipitates and WCE were immunoblotted with the indicated antibodies. ( f ) Forty-eight hours after transfection with the indicated DNA constructs, 293T cells were lysed and subjected to F-actin fractionation. Fractions were analysed by immunoblotting with the indicated antibodies. ( g ) Forty-eight hours after transfection with the indicated siRNAs, 293T cells were lysed and subjected to F-actin fractionation assay. Fractions were analysed by immunoblotting with the indicated antibodies. Full-length blots in all panels are presented in Supplementary Fig. S7 . Full size image Novel actin K84me1 regulates ALKBH4–actomyosin interaction A previously reported two-dimensional gel-electrophoresis approach, followed by immunoblotting using a pan-reactive anti-methyl-lysine mouse monoclonal antibody, revealed the existence of lysine-methylated actin proteins. However, no exact sites were identified [16] . Interestingly, the mass spectrometric analysis of ALKBH4 interacting proteins indicates that monomethylated actin (K84me1) was pulled down with ALKBH4 ( Supplementary Table S1 ). To further validate and investigate this observation, we generated an actin-K84me1 antibody that specifically recognizes K84-monomethylated actin ( Supplementary Fig. S2b ). We then purified HA-β-actin from human 293T cells, digested with Asp-N/Arg-C and enriched for potential K84me1 species by peptide immunoprecipitation using the actin-K84me1 antibody, and analysed by mass spectrometry. This mass spectrometry analysis confirmed that actin is indeed methylated on K84 ( Supplementary Fig. S2c,d and Supplementary Table S2 ). We then speculated that ALKBH4 might specifically interact with actin K84me1 and/or actin K84me1 might be an in vivo substrate of ALKBH4. By employing two different methylation-deficient actin mutants (K84A and K84R), we confirmed that actin is methylated on lysine 84 in vivo ( Fig. 2c ). We next examined the methylation profile between F-actin and G-actin in 293T cells. Interestingly, we found that under untreated conditions methylated actin preferentially exists as F-actin ( Fig. 2d , lanes 1, 2). After forced disassembly of F-actin into G-actin by F-actin depolymerizing drug cytochalasin D (CCD), high levels of K84me1 G-actin were detected ( Fig. 2d , lanes 3, 4). This suggests that methylated actin rapidly polymerize into filaments under physiological conditions and/or that demethylation preferentially takes place after filament formation. The expected shift in the F/G-actin ratio following treatment with either CCD ( Fig. 2d , lanes 3, 4) or the F-actin stabilizing drug phalloidin ( Fig. 2d , lanes 5, 6) confirmed efficient fractionation. Immunoblot analyses revealed that substitution of lysine 84 to arginine or alanine or treatment with the global methylation inhibitor AdOx (adenosine-2′, 3′-dialdehyde) abolished the actin–ALKBH4 interaction ( Figs 2e , 3g and Supplementary Fig. S3a,b ). This demonstrates that methylation of actin is required for efficient binding to ALKBH4. Mutation of lysine 84 to arginine and especially alanine results in a dramatic charge change that could impact the overall properties of actin. To determine if the mutants had retained functionality we tested their ability to polymerize into actin filaments. The F/G-actin fractionation showed that the distribution of G-actin and F-actin were similar in WT, K84A and K84R cells, demonstrating that both mutants could be readily incorporated into actin filaments in vivo ( Fig. 2f ). This is consistent with previous findings in yeast, showing that the K84A mutation had no effect on polymerization [37] . Furthermore, AdOx treatment did not affect actin’s ability to form filaments ( Supplementary Fig. S3c ). In accordance with our previous data showing a strong interaction between ALKBH4 and actin as well as a clear co-localization of ALKBH4 with F-actin, we observed that, though most ALKBH4 was found in the soluble fraction, a fraction of ALKBH4 sedimented into the insoluble fraction with F-actin ( Fig. 2g ). 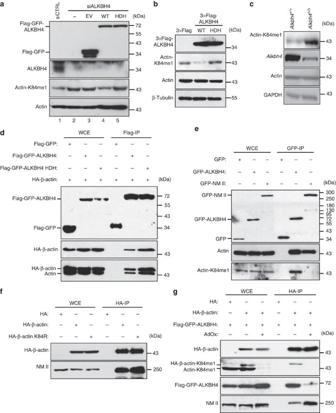Figure 3: ALKBH4 mediates demethylation of K84me1 actinin vivoregulating actomyosin interaction. (a) U2OS cells were simultaneously transfected with siCTRL or ALKBH4 siRNA, together with the indicated siRNA insensitive Flag-GFP-ALKBH4 constructs lysed, 48 h later cells were analysed by immunoblotting analysis using the indicated antibodies. (b) U2OS cells were transfected with WT or catalytically inactive ALKBH4 (HDH) and lysates were immunoblotted with the indicated antibodies. (c) ControlAlkbh4+/+Cre(Alkbh4+/+) andAlkbh4L/LCreMEF (Alkbh4Δ/Δ) cells were lysed and analysed by immunoblotting with the indicated antibodies. (d) 293T cells were co-transfected with Flag-GFP-ALKBH4 WT or HDH and HA-β-actin as indicated and lysates were subjected to Flag immunoprecipitation and immunoblotted with the indicated antibodies. (e) 293T/GFP-NM II or 293T/GFP-ALKBH4 stable cell lysates were subjected to GFP immunoprecipitation. Immunoprecipitates and WCEs were immunoblotted with the indicated antibodies. (f) 293T cells were transfected with WT or K84R HA-β-actin as indicated and lysates were subjected to HA immunoprecipitation. Immunoprecipitates and WCEs were immunoblotted with the indicated antibodies. Quantification of signal intensity of K84R relative to WT. (g) Forty-eight hours after transfection with the indicated DNA constructs, 293T cells were treated with 20 μM AdOx (adenosine-2′, 3′-dialdehyde) for 24 h, lysed and subjected to HA immunoprecipitation. Immunoprecipitates were analysed by immunoblotting with the indicated antibodies. Full-length blots in all panels are presented inSupplementary Fig. S7. Figure 3: ALKBH4 mediates demethylation of K84me1 actin in vivo regulating actomyosin interaction. ( a ) U2OS cells were simultaneously transfected with siCTRL or ALKBH4 siRNA, together with the indicated siRNA insensitive Flag-GFP-ALKBH4 constructs lysed, 48 h later cells were analysed by immunoblotting analysis using the indicated antibodies. ( b ) U2OS cells were transfected with WT or catalytically inactive ALKBH4 (HDH) and lysates were immunoblotted with the indicated antibodies. ( c ) Control Alkbh4 +/+ Cre ( Alkbh4 +/+ ) and Alkbh4 L/L Cre MEF ( Alkbh4 Δ/Δ ) cells were lysed and analysed by immunoblotting with the indicated antibodies. ( d ) 293T cells were co-transfected with Flag-GFP-ALKBH4 WT or HDH and HA-β-actin as indicated and lysates were subjected to Flag immunoprecipitation and immunoblotted with the indicated antibodies. ( e ) 293T/GFP-NM II or 293T/GFP-ALKBH4 stable cell lysates were subjected to GFP immunoprecipitation. Immunoprecipitates and WCEs were immunoblotted with the indicated antibodies. ( f ) 293T cells were transfected with WT or K84R HA-β-actin as indicated and lysates were subjected to HA immunoprecipitation. Immunoprecipitates and WCEs were immunoblotted with the indicated antibodies. Quantification of signal intensity of K84R relative to WT. ( g ) Forty-eight hours after transfection with the indicated DNA constructs, 293T cells were treated with 20 μM AdOx (adenosine-2′, 3′-dialdehyde) for 24 h, lysed and subjected to HA immunoprecipitation. Immunoprecipitates were analysed by immunoblotting with the indicated antibodies. Full-length blots in all panels are presented in Supplementary Fig. S7 . Full size image ALKBH4 promotes actin-NM II binding via actin demethylation Though no natural substrate for ALKBH4 has yet been described, we reasoned that as ALKBH4 binds to methylated actin, accumulates at the contractile ring and midbody during cytokinesis, and possesses dioxygenase activity in vitro [34] , ALKBH4 might mediate the removal of the methyl group on actin K84. To test this hypothesis, we first investigated if the level of actin-K84me1 correlated with expression of ALKBH4. Indeed, ALKBH4 depletion was accompanied by a dramatic increase in actin-K84me1 ( Fig. 3a , lane 1 versus 2). Importantly, the increase in methylation was completely prevented by complementation with WT ALKBH4, but not by ALKBH4 containing a mutated catalytic domain (H169A/D171A/H254A (HDH)) ( Fig. 3a , lanes 3–5). Additionally, overexpression of WT ALKBH4 but not the HDH ALKBH4 mutant resulted in a decrease in actin-K84me1 ( Fig. 3b ). Consistent with our findings in human cells, 4-hydroxytamoxifen (4-OHT) treatment of Alkbh4 L/L MEF cells (designated Alkbh4 Δ/Δ ) resulted in depletion of ALKBH4 and a pronounced increase in actin methylation ( Fig. 3c ). It has previously been observed that a substrate may not readily dissociate from a catalytically inactive enzyme [38] . In accordance with this and the possibility of actin being an ALKBH4 substrate, we observed that the actin–ALKBH4 interaction was stronger after disruption of the dioxygenase domain in ALKBH4 ( Fig. 3d ). These different independent pieces of in vivo data presented above makes a strong indication that the actin K84me1 demethylation is dependent on ALKBH4. X-ray crystallography and NMR have previously been used to predict the region of actin that binds to NM II (ref. 39 ). Interestingly, actin K84 is located within the predicted NM II interacting region, which made us speculate that methylation of K84 may influence the actin-NM II interaction. Intriguingly, and in contrast to ALKBH4 that preferentially binds to methylated actin, NM II does not interact with K84me1 ( Fig. 3e ). Furthermore, employing a methylation-deficient actin mutant, K84R, or inhibiting methylation by AdOx both resulted in increased NM II–actin interaction ( Fig. 3f and Supplementary Fig. S3b,d ), suggesting that ALKBH4-dependent demethylation of actin-K84me1 promotes binding of NM II to F-actin in the actomyosin network. The ALKBH4–actomyosin interaction is mediated by actin To better understand the functional interplay between components of the actomyosin network, we tested how depletion or inhibition of one component would affect the interaction of the other two. Consistent with the data that non-methylated actin interacts better with NM II, the NM II–actin interaction was greatly decreased in both ALKBH4-deficient MEF cells and human cells ( Fig. 4a ). NM II depletion did not influence the binding of ALKBH4 to actin ( Fig. 4c and Supplementary Fig. S3e ). Furthermore, treatment with the specific NM II inhibitor blebbistatin that inhibits myosin II’s ability to release phosphate and to bind tightly to actin filaments only affected the NM II–actin interaction but not the interaction between ALKBH4 and actin ( Fig. 4d and Supplementary Fig. S3f ) [40] . Due to the high cellular abundance of actin we could not achieve efficient actin depletion. However, CCD treatment significantly impaired the binding of NM II to both actin and ALKBH4 ( Fig. 4e and Supplementary Fig. S3g ), suggesting that filamentous actin mediates the interaction between ALKBH4 and NM II in the ALKBH4–actomyosin complex. This is also consistent with the observation that incubation with magnesium and ATP prevents co-precipitation of ALKBH4 and NM II ( Fig. 2a ). 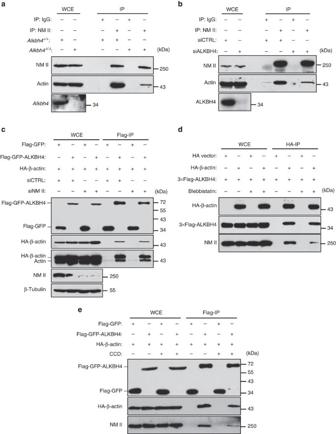Figure 4: The ALKBH4-Actomyosin interaction is mediated by actin. (a) Seventy-two hours after induction with 0.5 μM 4-OHT ControlAlkbh4+/+Cre(Alkbh4+/+) andAlkbh4L/LCre(Alkbh4Δ/Δ) MEF cells were lysed and subjected to NM II immunoprecipitation. Immunoprecipitates were analysed by immunoblotting with the indicated antibodies. (b) Forty-eight hours after transfection with the indicated siRNAs, 293T cells were lysed and subjected to NM II immunoprecipitation and subsequently immunoblotted with the indicated antibodies. (c) Forty-eight hours after transfection with the indicated siRNAs and DNA constructs, 293T cells were lysed and subjected to Flag immunoprecipitation. Immunoprecipitates were analysed by immunoblotting with the indicated antibodies. (d) Forty-eight hours after transfection with the indicated DNA constructs, 293T cells were treated with 5 μM Blebbistatin for 5 h, lysed and subjected to HA immunoprecipitation. Immunoprecipitates were analysed by immunoblotting with the indicated antibodies. (e) Forty-eight hours after transfection with the indicated DNA constructs, 293T cells were treated with 1 μg ml−1cytochalasin D (CCD) for 1.5 h, lysed and subjected to Flag immunoprecipitation. Immunoprecipitates were analysed by immunoblotting with the indicated antibodies. Full-length blots in all panels are presented inSupplementary Fig. S7. Figure 4: The ALKBH4-Actomyosin interaction is mediated by actin. ( a ) Seventy-two hours after induction with 0.5 μM 4-OHT Control Alkbh4 +/+ Cre ( Alkbh4 +/+ ) and Alkbh4 L/L Cre ( Alkbh4 Δ/Δ ) MEF cells were lysed and subjected to NM II immunoprecipitation. Immunoprecipitates were analysed by immunoblotting with the indicated antibodies. ( b ) Forty-eight hours after transfection with the indicated siRNAs, 293T cells were lysed and subjected to NM II immunoprecipitation and subsequently immunoblotted with the indicated antibodies. ( c ) Forty-eight hours after transfection with the indicated siRNAs and DNA constructs, 293T cells were lysed and subjected to Flag immunoprecipitation. Immunoprecipitates were analysed by immunoblotting with the indicated antibodies. ( d ) Forty-eight hours after transfection with the indicated DNA constructs, 293T cells were treated with 5 μM Blebbistatin for 5 h, lysed and subjected to HA immunoprecipitation. Immunoprecipitates were analysed by immunoblotting with the indicated antibodies. ( e ) Forty-eight hours after transfection with the indicated DNA constructs, 293T cells were treated with 1 μg ml −1 cytochalasin D (CCD) for 1.5 h, lysed and subjected to Flag immunoprecipitation. Immunoprecipitates were analysed by immunoblotting with the indicated antibodies. Full-length blots in all panels are presented in Supplementary Fig. S7 . Full size image ALKBH4 deficiency affects cleavage furrow organization The interaction of ALKBH4 with the actomyosin network and its ability to mediate demethylation of actin K84me1 suggest that ALKBH4 has an important role in cytokinesis. Strikingly, anillin and NM II failed to localize properly in ALKBH4-depleted cells during cytokinesis ( Fig. 5a ). The accumulation of the kinases Plk1 and aurora B at the midbody was also severely affected ( Fig. 5a and Supplementary Fig. S4a,b ), suggesting that ALKBH4-deficient cells have a defect in cleavage furrow formation. To investigate if ALKBH4 might also be important for other aspects of actomyosin dynamics than cytokinesis, we decided to study its impact on cell migration. Indeed, we observed a dramatic reduction in the migration ability of Alkbh4 Δ/Δ compared with Alkbh4 L/L MEF cells ( Fig. 5c and Supplementary Fig. S4c ), using the scratch assay method [41] . The cells were kept in low-serum medium to avoid proliferation and cell count after 24 h showed similar cell numbers between 4-OHT treated and untreated MEFs ( Supplementary Fig. S4d ). 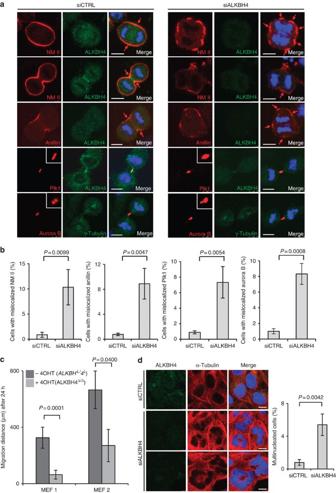Figure 5: ALKBH4 deficiency interferes with cleavage furrow organization and cell migration. (a) MRC5 cells were treated with ALKBH4 or CTRL siRNA for 48 h, fixed and immunostained with the indicated antibodies and DAPI. Scale bar, 10 μm. (b) Quantification of cells with mislocalised anillin, NM II, aurora B and Plk1 (shown ina). The histograms represent the mean of three independent experiments (500 cells per condition per experiment).P-values were calculated using a two-tailedt-test. Error bars indicate s.d. (c) Migration assays were performed with a monolayer of confluentAlkbh4Δ/ΔCreor control (Alkbh4L/LCre) MEF cells. The migration distances from the edges of the wound were calculated from the time point when the scratch was made (0 h) and 24 h later (illustrated inSupplementary Fig. S4c). Assays were run with primary MEFs derived from two different embryos.P-values were calculated using a two-tailedt-test. Error bars represent s.d. from multiple reading points. (d) MRC5 cells were treated with ALKBH4 or CTRL siRNA for 48 h, fixed and immunostained with the indicated antibodies and DAPI(left). Scale bar, 10 μm. Quantification of multinucleated cells (right). Histogram represents the mean of three independent experiments (500 cells per condition per experiment).P-values were calculated using a two-tailedt-test. Error bars indicate s.d. Figure 5: ALKBH4 deficiency interferes with cleavage furrow organization and cell migration. ( a ) MRC5 cells were treated with ALKBH4 or CTRL siRNA for 48 h, fixed and immunostained with the indicated antibodies and DAPI. Scale bar, 10 μm. ( b ) Quantification of cells with mislocalised anillin, NM II, aurora B and Plk1 (shown in a ). The histograms represent the mean of three independent experiments (500 cells per condition per experiment). P- values were calculated using a two-tailed t -test. Error bars indicate s.d. ( c ) Migration assays were performed with a monolayer of confluent Alkbh4 Δ/Δ Cre or control ( Alkbh4 L/L Cre ) MEF cells. The migration distances from the edges of the wound were calculated from the time point when the scratch was made (0 h) and 24 h later (illustrated in Supplementary Fig. S4c ). Assays were run with primary MEFs derived from two different embryos. P- values were calculated using a two-tailed t -test. Error bars represent s.d. from multiple reading points. ( d ) MRC5 cells were treated with ALKBH4 or CTRL siRNA for 48 h, fixed and immunostained with the indicated antibodies and DAPI(left). Scale bar, 10 μm. Quantification of multinucleated cells (right). Histogram represents the mean of three independent experiments (500 cells per condition per experiment). P- values were calculated using a two-tailed t -test. Error bars indicate s.d. Full size image Defects in the organization of the cleavage furrow may result in cytokinesis failure and formation of multinucleated cells. Indeed, ALKBH4-deficient cells, which exhibit clear defects in the organization of the cleavage furrow ( Fig. 5a ), also exhibited a dramatic increase in the frequency of multinucleation ( Fig. 5d and Supplementary Fig. S4e ). Multinucleated cells can result from cytokinesis failure or from a cell fusion event [42] . To distinguish between these possibilities, we followed cell division by live cell imaging, which confirmed that multinucleation observed after ALKBH4 depletion originated from aborted cytokinesis ( Supplementary Fig. S5a and Supplementary Movies 1 , 2 , 3 ). Importantly, ALKBH4-deficient cells required much longer time to exit mitosis ( Supplementary Fig. S5b ). In many cases, cytokinesis eventually failed resulting in refusion of the two new partly separated daughter cells or apoptosis. This is consistent with FACS analyses showing a significant increase in apoptosis and hyperploid cells following ALKBH4 depletion ( Fig. 6a and Supplementary Fig. S5c,d ). In addition, we observed that a portion of ALKBH4-depleted cells had more than two centrosomes ( Supplementary Fig. S6a ). The increase in centrosome number is likely a consequence of polyploidy caused by cells failing to go through cytokinesis. 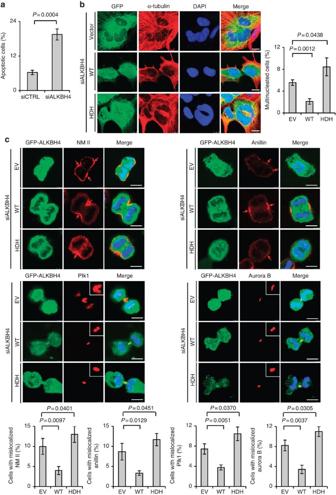Figure 6: Complementation with WT but not HDH ALKBH4 can rescue defects associated with cytokinesis failure. (a) Quantification of apoptotic cells (MRC5) following treatment with CTRL or ALKBH4 siRNA for 48 h. Quantification is based on three independent experiments (30,000 cells per condition per experiment).P-values were calculated using a two-tailedt-test. Error bars indicate s.d. (b) MRC5 cells were simultaneously treated with CTRL or ALKBH4 siRNA and the indicated siRNA insensitive Flag-GFP-ALKBH4 constructs for 48 h then analysed by immunofluorecence with the indicated antibodies. Quantification is based on three independent experiments (300 cells per condition per experiment).P-values were calculated using a two-tailedt-test. Error bars indicate s.d. (c) As in (b). Quantification of anillin, NM II, Plk1 and aurora B, mislocalization following treatment with CTRL or ALKBH4 siRNA and the indicated siRNA insensitive Flag-GFP-ALKBH4. Quantification is based on three independent experiments (300 cells per condition per experiment).P-values were calculated using a two-tailedt-test. Error bars indicate s.d. Figure 6: Complementation with WT but not HDH ALKBH4 can rescue defects associated with cytokinesis failure. ( a ) Quantification of apoptotic cells (MRC5) following treatment with CTRL or ALKBH4 siRNA for 48 h. Quantification is based on three independent experiments (30,000 cells per condition per experiment). P- values were calculated using a two-tailed t -test. Error bars indicate s.d. ( b ) MRC5 cells were simultaneously treated with CTRL or ALKBH4 siRNA and the indicated siRNA insensitive Flag-GFP-ALKBH4 constructs for 48 h then analysed by immunofluorecence with the indicated antibodies. Quantification is based on three independent experiments (300 cells per condition per experiment). P -values were calculated using a two-tailed t -test. Error bars indicate s.d. ( c ) As in ( b ). Quantification of anillin, NM II, Plk1 and aurora B, mislocalization following treatment with CTRL or ALKBH4 siRNA and the indicated siRNA insensitive Flag-GFP-ALKBH4. Quantification is based on three independent experiments (300 cells per condition per experiment). P- values were calculated using a two-tailed t -test. Error bars indicate s.d. Full size image Collectively, these data indicate that ALKBH4 depletion, in addition to impairing the function of the contractile ring and hence disorganize the cleavage furrow, most likely affect a broader range of actomyosin-related functions in the cell. Complementation with WT ALKBH4 rescues cytokinesis defects We next tested if reconstitution with WT and/or HDH-mutant ALKBH4 could rescue the cytokinesis-associated defects observed in ALKBH4-deficient cells. Cells were collected 48 h after simultaneous transfection with a combination of ALKBH4 small interfering RNA (siRNA) and ALKBH4 WT or ALKBH4 HDH. Complementation with WT, but not catalytically inactive ALKBH4, prevented multinucleation ( Fig. 6b and Supplementary Fig. S6b ) mislocalization of anillin, NM II, aurora B and Plk1 ( Fig. 6c ). Actually, overexpression of the HDH mutant in ALKBH4-depleted cells resulted in an even higher incidence of multinucleation ( Fig. 6b ) and cleavage furrow disorganization ( Fig. 6c ) compared with complementation with empty vector, suggesting that catalytically inactive ALKBH4 has a dominant-negative effect with regard to the ALKBH4 deficiency-associated phenotypes. In the present study, we have identified a novel post-translational modification on actin, K84 monomethylation, regulated by the previously uncharacterized dioxygenase ALKBH4. Though proteomic analysis using a pan-reactive anti-methyl lysine antibody previously suggested that actin might be methylated, no actual methylated residues were identified [16] . Our data demonstrate that ALKBH4-mediated demethylation of actin-K84me1 is important for maintaining actomyosin dynamics supporting normal cytokinesis and cell migration. It is not the first time PTMs of actin has been implicated in regulating cellular functions. Actin arginylation and H73me1 methylation have previously been proposed to regulate intracellular distribution of actin and polymer formation, respectively [43] , [44] . The interaction between the two major components of the actomyosin complex, actin and NM II, is regulated by ALKBH4-dependent demethylation of actin and is decreased in ALKBH4-deficient cells ( Fig. 4a ). These findings are further supported by the fact that NM II can bind more K84R mutant than WT actin ( Fig. 3f and Supplementary Fig. S3c ). In contrast, ALKBH4 specifically binds to the K84 methylated form of actin ( Fig. 2e and Fig. 3e ), and catalytically inactive ALKBH4 binds actin stronger than WT ( Fig. 3d ). We have attempted to test the in vitro demethylase activity of recombinant ALKBH4 or Flag-tagged ALKBH4 purified from human cells using either synthesized methylated peptide or HA-tagged β-actin purified from 293T cells. Unfortunately, these purified ALKBH4 proteins did not display vigorous demethylation/hydroxylation under any of the experimental settings examined. This most likely reflects a need for some unknown cofactors or that the F-actin conformation in the in vitro experiments is incompatible with efficient ALKBH4 demethylase activity. Despite the difficulties of showing in vitro activity of ALKBH4, the different independent in vivo data presented above makes actin a strong candidate substrate of the ALKBH4 dioxygenase activity. The reduced cell migration together with the severe problems associated with cytokinesis in ALKBH4-deficient human and murine cells suggest that ALKBH4-dependent demethylation of actin K84 has a very important role in regulating the actin–NM II interaction and actomyosin function. The facts that (1) cell motility and cytokinesis depend on proper actin–NM II interaction, (2) the actin–NM II interaction is compromised in ALKBH4-deficient cells and (3) NM II accumulation at the contractile ring and midbody is disturbed in ALKBH4-depleted cells, all point to a role of ALKBH4-mediated actin demethylation in promoting the recruitment of NM II to the cleavage furrow, and actin-NM II dependent structures in general. Actin fractionation revealed that, under physiological conditions, methylation of actin is preferentially observed on actin filaments and not monomeric actin. With regard to actomyosin dynamics in relation to cytokinesis our findings are consistent with the following model ( Fig. 7 ); upon recruitment to the contractile ring and midbody via interaction with methylated actin, ALKBH4 mediates demethylation of actin K84me1 and thus creates a binding site for NM II. Consecutive demethylation of actin moieties in the actin filament could then allow dynamic sliding of NM II along the actin filaments and mediate contraction of the contractile ring, resulting in cleavage furrow ingression and subsequent abscission. 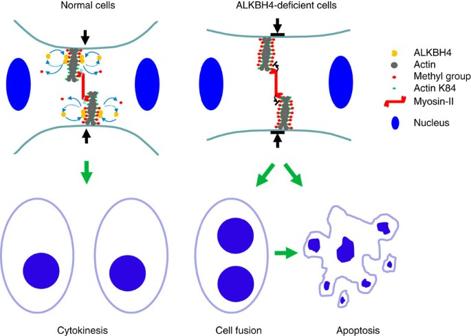Figure 7: Schematic model. The schematic describes a proposed model for the role of ALKBH4 in the regulation of actomyosin dynamics and cleavage furrow ingression during cytokinesis, and that ALKBH4 deficiency leads to cytokinesis failure or apoptosis (see discussion section for detailed explanation). Figure 7: Schematic model. The schematic describes a proposed model for the role of ALKBH4 in the regulation of actomyosin dynamics and cleavage furrow ingression during cytokinesis, and that ALKBH4 deficiency leads to cytokinesis failure or apoptosis (see discussion section for detailed explanation). Full size image Similarly to the previously described embryonic lethality of homozygous actin or NM II knock-out mice [45] , [46] , [47] , [48] , homozygous Alkbh4 knockout was also found to be embryonically lethal ( Fig. 1a ). This is in accordance with an essential function of ALKBH4 in regulating actomyosin function and supports our findings of an important role of ALKBH4 in cytokinesis. However, the fact that not all cells appear to have severe cytokinesis defects might suggest that ALKBH4-mediated actin demethylation and perhaps demethylation of yet unknown targets might be important not only for proper cytokinesis but for a far wider range of cellular functions. No homozygous actin deletions or nonsense mutations have been described in humans, probably because, like in mice, such deletions or mutations would be lethal. However, several missense mutations have been associated with human diseases including mental retardation and developmental malformations [49] , [50] , [51] . In mice, such mutations have been associated with tumourigenesis and metastasis [52] . Identification of ALKBH4 as a new regulator of actomyosin function opens up the possibility that ALKBH4 might also be targeted by mutations in developmental diseases and cancer. In conclusion, we propose that the key purpose of actin methylation and demethylation mediated by ALKBH4 is to create ‘handles’ for NM II, to ‘hold on to’ when ‘climbing’ along the actin filament thereby generating contraction of the actomyosin network ( Fig. 7 ). Plasmids and protein purification The human ALKBH4 gene was subcloned into p3 × flag-CMV14 (Sigma), pEGFP-c1b or pGEX-5x-2 (GE Healthcare) [53] . The human β-actin gene was subcloned into pcDNA3-HA (Invitrogen) and pCMV-GFP-MyoII-B was ordered from Addgene. Mutations were introduced using the QuickChange site-directed mutagenesis kit (Stratagene). Recombinant GST-ALKBH4 protein was expressed in E. coli strain BL21(DE3) and purified as described in the commercial available instructions. Cell culture and antibodies Human MRC5 and 293T cells were cultured in RPMI 1640 at 37 °C, 5% CO2 with 10% fetal bovine serum and 1% (w/v) penicillin/streptomycin (Sigma). Human U2OS cells were grown in Dulbecco’s modified Eagle’s medium with 10% fetal bovine serum. Cells were treated with the following drugs: Nocodazole (Sigma), Cytochalasin D (Sigma) and Blebbistatin (Sigma) at the indicated periods of time and concentrations. The following antibodies were used in the study: Abcam: rabbit-anti-Histone H3 phosphor-S10, mouse-anti-p53, mouse-anti-myosin-II, mouse-anti-GAPDH. Invitrogen: F-actin (phalloidin-Texas Red). Sigma: mouse-anti-β-tubulin, mouse-anti-γ-tubulin, mouse-anti-α-tubulin, mouse-anti-actin, mouse-anti-flag, rabbit-anti-flag. Santa Cruz: rabbit polyclonal anti-actin, goat-anti-anillin, mouse-anti-Plk1. CWbiotech: rabbit-anti-HA, mouse-anti-GFP. Bethyl: rabbit-anti-aurora B. ALKBH4: no. 1, generated using purified recombinant GST-ALKBH4 protein (AbMax Biotechnology), ALKBH4: no. 2 generated using human synthetic peptide (101QSGRKKQDYGPK112) (CWbiotech). Rabbit polyclonal anti-actin K84-monomethylated antibody (anti-actin K84me1) was generated using a synthetic peptide with monomethylated lysine 84 (77TNWDDMEm K IWHHTFY91) as immunogen (New England Peptide, Boston, USA). Plasmid transfection and RNA interference DNA transfections were carried out using polyetylenimine or Lipofectamine 2000 (Invitrogen). siRNA duplexes (GenePharma, China) were transfected into cells using Lipofectamine RNAiMAX (Invitrogen) according to the manufacturer’s instructions. For ALKBH4 rescue experiments, cells were co-transfected with 1 μg of plasmid DNA and 60 pmol siRNA using Lipofectamine 2000. The following siRNA sequences were used in the study: ALKBH4 no. 1: 5′-GAUCCCGGGAUUGAAAUGA-3′, ALKBH4 no. 2: 5′-GGGAUUGAAAUGAGGAGCA-3′, ALKBH4 no. 3: 5′-GGGAUCAUUUGAGCUUAAA-3′. NM II no. 1: 5′-GGGCCAACAUUGAAACAUA-3′, NM II no. 2: 5′-GUGCUACAGUUUGGAAATA-3′, NM II n3: 5′-CUCGGGAUGAGGUGAUUAA-3′, Scrambled siRNA (siCTRL): 5′-UUCUCCGAACGUGUCACGU-3′. Immunofluorescence analysis Cells seeded onto coverslips were fixed with methanol or 4% paraformaldehyde on ice, then permeabilized with 0.1% Triton X-100 and 0.05% NP-40 on ice. After pre-blocking the coverslips were first incubated with primary antibody, then fluorescent dye-conjugated secondary antibody and mounted with DAPI-containing mounting medium (Vector Laboratories, Burlingame, CA). Confocal images were acquired and analysed on Leica TCS SP5 (Leica) equipped with HCX PL APO 63 × 1.4 oil CS immersion objective (Leica). Immunoprecipitation Whole-cell extract was generated by lysing cells in NET buffer (50 mM Tris-HCl pH7.4, 150 mM NaCl, 5 mM EDTA, 0.1% NP-40 and protease inhibitors) followed by sonication using a SonicDismembrator (Fisher Scientific) (1 min, with 10 s-on and 20 s-off cycles). When using CCD treatment, CCD was added to the NET buffer. Anti-Flag M2 affinity gel (Sigma), anti-HA affinity gel (Sigma) and anti-GFP-Trap-A beads (ChromoTek) were used for immunoprecipitations. Identification of methylation sites by mass spectrometry HA-tagged β-actin was immunoprecipitated from 293T cells 48 h after transfection, eluted from the beads with 100 mM glycine pH 2.5, and immediately neutralized with Tris buffer. The proteins were then precipitated with four volumes of cold acetone, air dried and resuspended in 8 M urea, 100 mM Tris, pH 8.5. After reduction (5 mM TCEP, 20 min, RT ) and alkylation (10 mM iodoacetamide, 15 min, RT), the sample was diluted to 2 M urea, 100 mM Tris pH 8.5, followed by Asp-N (Roche, Cat. No. 11420488001) digestion (1:50 enzyme:substrate, 37 °C, O/N), Asp-N inactivation (0.5 mM EDTA for 2 min), and Arg-C (Roche, Cat. No. 11370529001) digestion (1:50 enzyme:substrate, 37 °C, 8 h with 5 mM DTT and 8.5 mM CaCl 2 ). The digestion was quenched with 5% formic acid and the peptides were desalted and re-dissolved in the NET buffer. Methylated β-actin peptides were further enriched by IP using actin K84me1 antibody. After elution (with 100 mM glycine, pH 2.5) and desalting, the enriched peptides were analysed on an Easy-nLC 1000 UPLC (Thermo Fisher Scientific) coupled to a Q Exactive mass spectrometer (Thermo Fisher Scientific). Peptides were loaded on a pre-column (75 μm ID packed with 8 cm 10 μm-C18 resin) and separated on an analytical 75 μm ID column packed with 11 cm 3 μm-C18 resin (pre-column: ODS-AQ 12 nM S-10 μm (YMC Co., Ltd), analytical column: Luna 3 μm 100 Å resin ( Phenomenex )) with anacetonitrile gradient from 0–25% in 60 min and 25–80% in another 7 min at a flow rate of 200 nl min −1 . Spectra were acquired in a data-dependent mode: the 10 most intense ions of +2, +3 or +4 charge from each full scan ( R =70,000) were isolated for HCD MS2 ( R =17,500) at NEC 27 with a dynamic exclusion time of 150 s. For peptide identification, the MS2 spectra were searched against an EPI-IPI human database (forward+reversed sequences) using Prolucid with 50 p.p.m. mass accuracy for both precursor and fragment ions and considering carbamidomethylation on Cys as a fixed modification and mono-, di- or tri-methylation at Lys as differential modifications [54] . Search results were filtered using DTASelect 2.0 with 10 p.p.m. mass accuracy for precursor mass and a 1% FDR cutoff at the spectral level [55] . The β-actin K84me1 spectra presented in the figures were annotated using pLabel, requiring 20 p.p.m. accuracy for fragment ions [56] . The data files have been uploaded to http://www.peptideatlas.org/ with the access number: PASS00132 and password: WW685h. Time-lapse microscopy Cells were placed in a 37 °C heated microscope chamber and observed under differential interference contrast. Images were acquired every 2 min with Olympus IX81 microscope, equipped with Olympus × 40 dry lens and processed using Andor iQ2.7 image browser software. FACS analyses For cell cycle analysis the Cycle test Plus DNA reagent kit was applied according to the manufacturer’s instructions (Becton-Dickinson). FACS analysis was carried out on a FACSAria III equipped with FACSDiva software 6.0 (Becton-Dickinson) and Modfit LT software (version 3.1, BD). Apoptotic cells were detected by staining with annexin-PI using the Annexin V-FITC and PI Apoptosis Detection Kit (Jiamay Biotech) and analysed by flow cytometry. Midbody isolation Midbody purification was performed according to the protocol developed by Mullins and McIntosh and Sellitto and Kuriyama [57] , [58] . F-actin fractionation assay The ratio of F-actin versus G-actin in cells was analysed using an F-actin/G-actin in vivo assay kit (Cytoskeleton) based on the manufacturer’s protocol. Generation of conditionally targeted Alkbh4 mice Gene targeting vector containing ALKBH4 exon 2 and exon 3 was constructed by cloning genomic ALKBH4 fragments into the pCR4-TOPO vector (Invitrogen) from BAC clone bMQ 337L22 BAC clone (Geneservice). Two LoxP sites were inserted, flanking an inserted neomycin-resistance gene cassette and the exon 2 and exon 3 regions. A Diphteria Toxin A ( DTA ) gene was used for negative selection. The targeting vector was linearized with Nru I and electroporated into 129Sv/Pas ES cells. ES cells were selected with 200 μg ml −1 G418. Positive ES cell clones were injected into C57BL/6N blastocysts. Chimeric mice ( Alkbh4 +/L ) were crossed with a C56BL/6 Cre-deleter mouse strain (GenOway) to generate heterozygous conventional knock-out mice. Southern blotting assay Genomic DNA was digested with Spe I/ Pci I and hybridized using an external 524 bp probe (Ext 5′probe) located upstream of the 5′ homology sequence and an internal 399 bp probe (Int 3′probe) located within the 3′ homology sequence of the targeting vector. Pre-hybridization and hybridization: 4 × SSC, 1% SDS, 0.5% skimmed milk, 20 mM EDTA, 100 μg ml −1 hering sperm, at 65 °C for 18 h. Washings: two times 3 × SSC, 1% SDS at 65 °C for 15 min, then two times 0.5 × SSC, 1% SDS at 65 °C for 15 min. Primers used: external 5′ probe: 5′-TCGCTAAGGCCCGCTGCCGGGGAGC-3′ and 5′-AAATGCAGAGATCTCGGCGT-3′. Internal 3′ probe: 5′-TAGTACAGGCTGGCCTCAAAAT-3′ and 5′-ATCACCAGAACCACCATGAGG-3′. Isolation and culture of MEFs Mice homozygous for the recombined allele ( Alkbh4 L/L ) were bred with a mouse line ubiquitously expressing the Cre-ER transgene (mouseline: B6. Cg-Tg (CAG-cre/Esr1) 5 Amc J −1 , Jackson Laboratory), inducible by tamoxifen, to generate Alkbh4 L/L Cre mouse strain. MEFs were isolated from 12.5–13.5 dpc embryos according to protocol described [59] , and grown in Dulbeccos modified Eagle’s medium supplemented with 10% fetal calf serum, 1% GlutaMAX (Invitrogen) and 1% PenStrep (Invitrogen). Alkbh4 deletion in Alkbh4 L/L Cre cell lines was accomplished by 0.5 μM 4-hydroxytamoxifen (4-OHT, Sigma H6278) treatment in MEF culture medium for 4 days. Alkbh4 +/+ Cre primary MEF cell lines were used as control cells for the experiments. Primary MEF cell lines (up to passage 5) were used in the experiments. Cell scratch assay The migration assay was performed as described [41] . Cell counting experiments were performed by plating equal numbers (10 5 ) of primary Alkbh4 L/L Cre MEFs, treated or untreated with 4-OHT in each well of six-well plates containing low-serum medium (0.5% FBS), and the cells were counted every 24 h using a hemocytometer. Genotyping Mice were PCR genotyped with the following primer sets: WT allele (+), Alkbh4-2+ and Alkbh4-4- (340 bp); recombined allele (L), Alkbh4-2+ and Alkbh4-NEO (1,003 bp); knock-out allele (−) or Cre-ER-mediated ΔL, Alkbh4-2+ and Alkbh4-2- (550 bp). Expand long template kit PCR kit (Roche) was used with 10 pmol forward and reverse primers. Primer sequences: Alkbh4-2+: 5′-AGTTGCTTTAGTTCCAAGAAGAGCATCGG-3′, Alkbh4-2-: 5′-GCCTCCCAAAACTTGGTATCACAAACC-3′, Alkbh4-4-: 5′-TGAGCTGCTGACGTGCTTAACC-3′, Alkbh4-NEO-: 5′-TCTCACCTTGCTCCTGCCGAGAAAGTATC-3′. Statistical analysis Two-tailed t -tests in grouped analyses of Prism5 software were applied. P -value <0.05 was considered significant. Accession codes: Mass spectrometry data have been uploaded to Peptide Atlas under accession code PASS00132. How to cite this article: Li, M.-M. et al . ALKBH4-dependent demethylation of actin regulates actomyosin dynamics. Nat. Commun. 4:1832 doi: 10.1038/ncomms2863 (2013).